Ants and termites increase crop yield in a dry climate Agricultural intensification has increased crop yields, but at high economic and environmental cost. Harnessing ecosystem services of naturally occurring organisms is a cheaper but under-appreciated approach, because the functional roles of organisms are not linked to crop yields, especially outside the northern temperate zone. Ecosystem services in soil come from earthworms in these cooler and wetter latitudes; what may fulfill their functional role in agriculture in warmer and drier habitats, where they are absent, is unproven. Here we show in a field experiment that ants and termites increase wheat yield by 36% from increased soil water infiltration due to their tunnels and improved soil nitrogen. Our results suggest that ants and termites have similar functional roles to earthworms, and that they may provide valuable ecosystem services in dryland agriculture, which may become increasingly important for agricultural sustainability in arid climates. The agricultural intensification known as the 'green revolution' has dramatically increased crop yields, but it is questionable whether intensive practices are sustainable in the long term [1] , [2] , [3] , [4] . There are the increasing costs of petroleum-based products such as herbicides, pesticides, fertilizers and energy inputs, and increasing costs of water. In addition, agricultural intensification has caused environmental degradation from loss of biodiversity due to monoculture of agriculturally important species, loss and fragmentation of habitat, chemical inputs into waterways and deterioration of soil health [4] , [5] , [6] . One approach to developing more sustainable agriculture is to maintain or restore natural ecosystem services that reduce dependence on human inputs to agricultural systems [6] , [7] , [8] . Examples of ecosystem services used in agriculture are dung burial [9] , pollination [10] and predation or parasitism, to reduce insect herbivores by natural enemies or 'beneficial insects' [11] , [12] . Earthworms are well known to improve soil health in both native and agricultural systems [13] , [14] , and are considered to be 'ecosystem engineers' [15] . Earthworms affect soil structure by increasing porosity and decreasing bulk density, both of which lead to greater water infiltration into the soil, and they can also increase the supply of nitrogen and other nutrients [13] , [14] . As a consequence, earthworms have been shown to increase plant growth [16] , [17] , but their role in intensive agricultural production systems is limited by excessive soil disturbance. Lower-intensity farm management practices have been developed to reduce erosion, soil compaction, carbon loss, evaporation from the soil and reduction of synthetic chemical input. Collectively, these practices are referred to as 'conservation agriculture', and include practices such as reduced tillage [18] , [19] , [20] , direct drilling [21] for seeding (to reduce soil disturbance), physical weed control (that is, shallow tillage) [22] and controlled traffic [23] . These practices were found to conserve earthworms and are now promoted for this purpose as well [13] , [24] . Earthworms are limited in their distribution to wetter and cooler habitats [13] , [14] . Ants and termites appear to replace earthworms as soil ecosystem engineers in drier and hotter habitats [15] , [25] , [26] , [27] , [28] . Various studies have shown that ants and termites help to create soil structure, influence aeration, water infiltration and nutrient cycling in natural ecosystems [27] , [28] , [29] . However, despite the apparent similarity in functional roles in soil that ants and termites have with earthworms, their potential use in intensive agriculture in drier and hotter habitats has been largely overlooked. Furthermore, despite widespread acknowledgement of the importance of biodiversity on ecosystem services [7] , [8] , [11] , [12] and small-scale demonstration of the link between soil faunal activity and plant growth in microcosms [17] , [30] , there has been no experimental field-scale demonstration of a direct positive relationship between a rich soil macrofauna and enhanced crop yield in sustainable agriculture [13] , [14] , [16] , [17] , [30] . In this study, we tested whether the presence of ants and termites affects crop yield, and investigated the mechanism by which that effect occurs. We conducted an experiment on a farm with some conservation agriculture management and, therefore, diverse soil fauna. We chose this farm partly because it lies near the arid extreme of wheat production in Australia [31] , and partly because earthworms are absent [32] (thus, the effects can be attributed to ants and termites). We excluded ants and termites and measured the impacts of ant and termite activity and crop yield over 3 years; we also tilled to mimic physical weed control to determine its effect on ant and termite activity. We investigated the two major mechanisms by which these insects might affect crop yield: soil macropores, the channels through soil that increase water infiltration [15] , [16] , [26] , [27] , [28] (here, insect tunnels), and soil nutrients, as soil fauna transform these nutrients from organic to mineral forms, which can be assimilated by plants [16] , [25] , [26] , [27] , [28] , [29] , [30] . We predicted that the exclusion treatment would reduce soil tunnels, and hence reduce soil moisture infiltration during rainfall events, and also reduce mineral soil nutrients over time. We found that ants and termites raise crop yield by increasing water infiltration into the soil through their tunnels and by increasing the supply of soil mineral nitrogen. Results from this study have provided the first demonstration that the presence of ants and termites raise crop yield by contributing valuable ecosystem services, and hence may become a new tool for sustainable management of production landscapes in drier climates. As the arid conditions of the experiment mimic future temperature and rainfall conditions of many of the major wheat production areas predicted under climate change, these results may be pertinent for climate adaptation. Exclusion efficacy We excluded ants and termites from half the experimental plots (27×27 m 2 , Supplementary Fig. S1a ; sized to be relevant for foraging distances of ants and termites) using liquid insecticide ( Supplementary Figs. S1b and S2a ) and tilled half the experimental plots to mimic physical weed control (15 cm deep; Supplementary Figs. S1b and S2b ). All plots had similar numbers of active ant nests before treatment (exclusion: F 1,16 =0.008, P =0.932; tillage: F 1,16 =0.190, P =0.669; exclusion × tillage interaction: F 1,16 =0.274, P =0.608), whereas at harvest (6 months after application of the exclusion treatment), the exclusion plots had an 85% reduction in active ant nests compared with water control plots. Tillage (no-till versus tilled) and the tillage × exclusion interaction were not significant (exclusion: F 1,16 =76.180, P <0.001; tillage: F 1,16 =0.569, P =0.462; exclusion × tillage interaction: F 1,16 =0.418, P =0.527; Supplementary Table S1 ; Fig. 1a ). Termite contact with and its presence in baits was around twice as high in control plots compared with exclusion plots, again tillage was not significant (exclusion: F 1,16 =13.635, P =0.002; tillage: F 1,16 =0.070, P =0.795; exclusion × tillage interaction: F 1,16 =0.278, P =0.605; Supplementary Table S2 ; Fig. 1b ). Grass-eating termite species (especially Amitermes and Drepanotermes species), presumably eating the wheat stubble, were only found in control plots, whereas wood-eating species (mostly Microcerotermes species), surviving on tree roots from the cleared native vegetation, were found in exclusion plots as well. 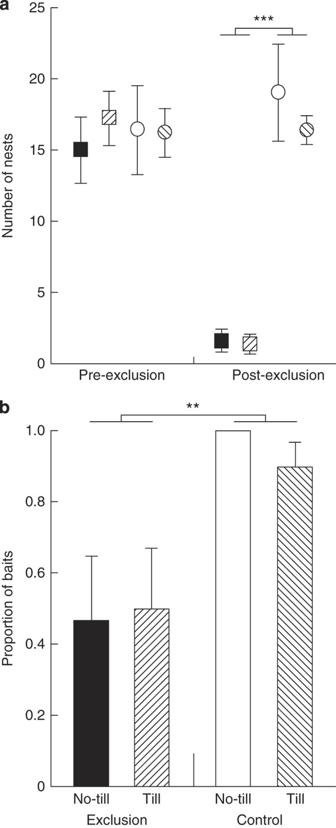Figure 1: Efficacy of exclusion treatment. Effect was measured as (a) number of active ant nests per plot, pre-exclusion (at sowing May 2006) and post-exclusion (at harvest November 2006); ***P<0.001,n=5 and (b) number of baits contacted by termites post-exclusion (pre-sowing 2008); **P=0.002,n=5. Data are means±standard errors; exclusion plots are squares, control plots are circles, tilled plots are hatched, no-till plots are solid colours. Figure 1: Efficacy of exclusion treatment. Effect was measured as ( a ) number of active ant nests per plot, pre-exclusion (at sowing May 2006) and post-exclusion (at harvest November 2006); *** P <0.001, n =5 and ( b ) number of baits contacted by termites post-exclusion (pre-sowing 2008); ** P =0.002, n =5. Data are means±standard errors; exclusion plots are squares, control plots are circles, tilled plots are hatched, no-till plots are solid colours. Full size image Crop yield There were two crop harvests, in November 2006 (6 months after application of the exclusion treatment) and in November 2008 (fallow years such as 2007 are used to accumulate soil moisture). Wheat yield was higher in 2006 (3.51±0.09 t ha −1 ) than in 2008 (2.11±0.07 t ha −1 ; year: F 1,16 =128.161, P <0.001; Supplementary Table S3 ), driven by water availability (cumulative rainfall at seeding in 2006 was 429 mm and in 2008 was 361 mm; Supplementary Fig. S3 ). This was confirmed by the threefold increase of small and incompletely filled ('pinched') kernels, which did not differ between treatments, but was significantly different between years (exclusion: F 1,16 =0.192, P =0.667; tillage: F 1,16 <0.001, P =0.989; exclusion × tillage interaction, F 1,16 =0.089, P =0.789; year, F 1,16 =61.303, P <0.001; all year interactions were not significant; Supplementary Table S4 ; Fig. 2a ). There were no differences in wheat yield between treatments in 2006 (exclusion: F 1,16 =0.367, P =0.553; tillage: F 1,16 =0.175, P =0.681; exclusion × tillage interaction: F 1,16 =0.224, P =0.642), but in 2008, wheat yield was on average 36% higher in control compared with exclusion plots (exclusion: F 1,16 =10.620, P =0.005) and on average 15% higher (but nonsignificant) in tilled compared with no-till plots (tillage: F 1,16 =2.632, P =0.124; exclusion × tillage interaction: F 1,16 =0.241, P =0.630; Supplementary Table S5 ; Fig. 2b ). 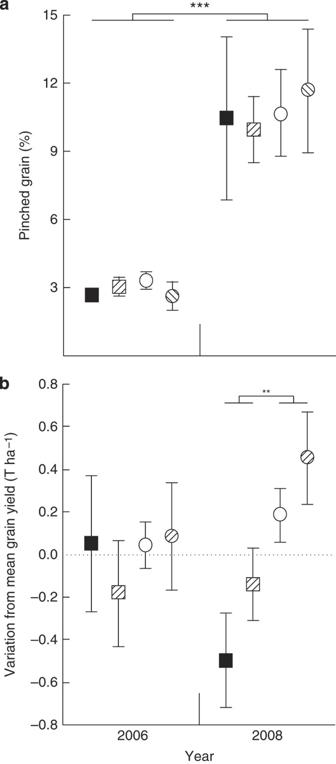Figure 2: Crop yield in plots with or without soil insects and tillage. Yield was measured in 2006, when treatments were applied, and in 2008. (a) Pinched grain as percentage of total weight; ***P<0.001,n=5. (b) Variation from average wheat yield. Data are means±standard errors; exclusion plots are squares, control plots are circles, tilled plots are hatched, no-till plots are solid colours; **P=0.005,n=5. Figure 2: Crop yield in plots with or without soil insects and tillage. Yield was measured in 2006, when treatments were applied, and in 2008. ( a ) Pinched grain as percentage of total weight; *** P <0.001, n =5. ( b ) Variation from average wheat yield. Data are means±standard errors; exclusion plots are squares, control plots are circles, tilled plots are hatched, no-till plots are solid colours; ** P =0.005, n =5. Full size image Insect tunnels There were the same numbers of insect tunnels (0.65 per 100 cm 2 ) in the plots during various treatments in 2006. In 2008, there were more insect tunnels in control (0.7 per 100 cm 2 ) than in exclusion plots (0.35 per 100 cm 2 ; exclusion: F 1,16 =12.457, P =0.003), and tillage was not significant (tillage: F 1,16 =1.769, P =0.202; exclusion × tillage interaction: F 1,16 =0.597, P =0.451; Supplementary Table S6 ; Fig. 3 ). This change with time indicates that the insecticide killed the insects in 2006, but the tunnels only collapsed slowly over time without maintenance so that by 2008, there were 50% fewer tunnels in the exclusion plots. 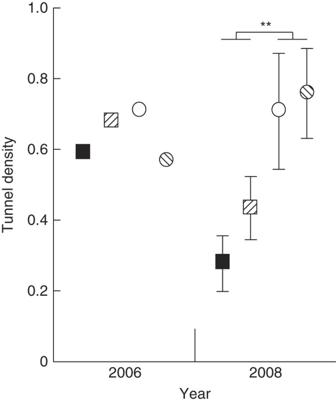Figure 3: Tunnel density in soil with or without soil insects and tillage. Data are mean number of ant and termite tunnels per 100 cm2(±standard errors) after harvest in 2006 (n=1) and after harvest in 2008 (n=5); **P=0.003. Exclusion plots are squares, control plots are circles, tilled plots are hatched and no-till plots are solid colours. Figure 3: Tunnel density in soil with or without soil insects and tillage. Data are mean number of ant and termite tunnels per 100 cm 2 (±standard errors) after harvest in 2006 ( n =1) and after harvest in 2008 ( n =5); ** P =0.003. Exclusion plots are squares, control plots are circles, tilled plots are hatched and no-till plots are solid colours. Full size image Water infiltration In 2006, the increase in soil moisture at a depth of 50 cm during rainfall did not differ significantly between treatments (exclusion: F 1,12 =0.174, P =0.684; tillage: F 1,12 =1.849, P =0.199; exclusion × tillage interaction, F 1,12 =2.174, P =0.166; Supplementary Table S7 ; Fig. 4a ). In 2008, soil moisture at 50 cm after an almost identical rainfall event increased three times more in control plots compared with exclusion plots (exclusion: F 1,12 =10.260, P =0.008), but there was no difference for tillage (tillage: F 1,12 =0.001, P =0.977; exclusion × tillage interaction: F 1,12 =0.019, P =0.892; Supplementary Table S7 ; Fig. 4b ). Compared with moisture at the surface, moisture at this depth is much less likely to evaporate from the soil and, therefore, is more likely to be used by plants for growth and grain production. 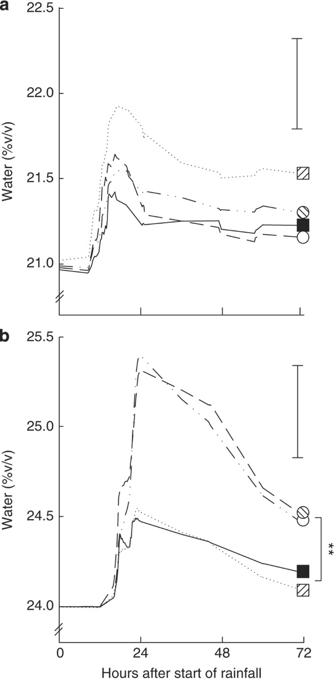Figure 4: Soil water content with or without soil insects and tillage. Soil water content at a depth of 50 cm was measured in plots with or without soil insects and tillage during similar rainfall events. In (a) 2006 (12 mm on 8 September) and (b) 2008 (11 mm on 9 June). Data are means, bars are least significant differences,n=5; **P=0.008. Exclusion plots are squares, control plots are circles, tilled plots are hatched and no-till plots are solid colours. Figure 4: Soil water content with or without soil insects and tillage. Soil water content at a depth of 50 cm was measured in plots with or without soil insects and tillage during similar rainfall events. In ( a ) 2006 (12 mm on 8 September) and ( b ) 2008 (11 mm on 9 June). Data are means, bars are least significant differences, n =5; ** P =0.008. Exclusion plots are squares, control plots are circles, tilled plots are hatched and no-till plots are solid colours. Full size image Soil mineral nitrogen The total mineral nitrogen in the soil after harvest in 2006 (12.6±1.4 mg kg −1 ) was higher than in 2008 (3.8±0.8 mg kg −1 ), reflecting time since last fertilizer application (year: F 1,16 =39.851, P <0.001; Supplementary Table S8 ). In 2006, there was no difference between treatments (exclusion: F 1,16 =3.348, P =0.086; tillage: F 1,16 =0.070, P =0.794; exclusion × tillage interaction: F 1,16 =0.183, P =0.674). In 2008, total mineral nitrogen in control plots was significantly higher than in exclusion (exclusion, F 1,16 =14.999, P =0.001), and there were no differences for tillage (tillage, F 1,16 =0.038, P =0.847; exclusion x tillage interaction: F 1,16 <0.001, P =0.985; Supplementary Table S9 ; Fig. 5 ). It appears that removal of soil macrofauna reduced total mineral nitrogen in exclusion plots by ∼ 70% compared with controls. Further evidence to support this suggestion comes from the variation in total mineral nitrogen. The variation in mineral nitrogen between plots within treatments was high in 2006 and in control plots in 2008, compared with exclusion plots in 2008. This variation is likely due to patches of high mineral nitrogen concentration, possibly in the thick walls of termite tunnels. Termites use a mixture of saliva and faeces to plaster their tunnel walls. The high level of nitrogen in termite faeces does not originate from their low nitrogen food sources (the cellulose of plant cell walls), but may have originated from the symbiotic gut bacteria that fix atmospheric nitrogen using the dinitrogenase reductase ( nifH ) gene [33] , [34] , which we found in the gut contents of termites collected from the field site. 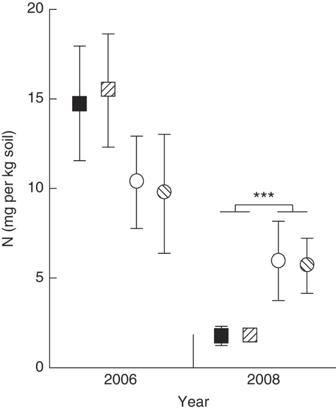Figure 5: Total mineral soil nitrogen in plots with or without soil insects and tillage. Data are means±standard errors measured after harvest in 2006 and after harvest in 2008;n=5, ***P=0.001. Exclusion plots are squares, control plots are circles, tilled plots are hatched and no-till plots are solid colours. Figure 5: Total mineral soil nitrogen in plots with or without soil insects and tillage. Data are means±standard errors measured after harvest in 2006 and after harvest in 2008; n =5, *** P =0.001. Exclusion plots are squares, control plots are circles, tilled plots are hatched and no-till plots are solid colours. Full size image This study demonstrates that ants and termites, the soil macrofauna in this dry and hot region, were associated with higher wheat crop yield under a low tillage, controlled traffic, but otherwise conventional agricultural management. We hypothesized two functional roles of the insects that could provide potential mechanisms to enhance yield, one of which was identified and a second was suggested in this study. The identified functional role was the digging of tunnels by the ants and the termites, which they do to forage and nest. These tunnels are a type of soil macropore [26] , [27] , [28] , [29] that allowed more rain water to infiltrate into the soil. Greater water infiltration deeper into the soil leads to lower evaporation from the soil surface, allowing plants a better access to the available water. It is also possible that greater infiltration leads to lower water run-off and erosion [35] . The second activity was the effect on mineral nitrogen by the insects in the soil. Although total mineral nitrogen declined overall, it did not decline as quickly in control compared with exclusion plots. In addition, as the yield was higher in the control plots, it seems likely that more nitrogen was removed from the soil by the wheat plants in these plots. If so, then the differences in mineral nitrogen in the soil between control and exclusion plots would have been greater than that measured. Although our understanding of the soil nitrogen cycle and how plants use soil nitrogen is developing [36] , there are several possible explanations for this effect: decreased mineralization, increased immobilization and increased denitrification. Another possibility is nitrogen fixation, normally associated with legumes [37] , but found in termites [33] , [34] , which has been implicated in native habitats [38] , [39] . We did not investigate all these possibilities, which can be influenced by abiotic or biotic factors [36] . We did, however, find evidence for nitrogen-fixing capacity by termites from the field. Whatever the exact mechanism, the presence of ants and the termites reduced the decline of total nitrogen by ∼ 9 mg kg −1 over the experiment, which corresponds to around 8 kg nitrogen per ha. This corresponds to 22–32% of the nitrogen typically added as urea fertilizer on farms in the region, suggesting that maintaining these soil macrofauna may help to lower fertilizer costs. The effects we found are large, and perhaps could have been predicted from the large impacts ants and termites are known to have on soil and biotic communities in natural habitats. They move tonnes of soil per hectare, increase aeration and influence availability of several nutrients [26] , [27] , [28] , [29] , [40] . They have direct and indirect effects on plants and herbivores and even indirect effects on predators in natural systems [41] , [42] , [43] , [44] ; hence, perhaps, it is not surprising that they had such a large impact in an agricultural system. Their impacts on natural ecosystems appear to be greatest in hot and seasonally dry climates [25] , [26] , [27] , [28] , [29] , similar to that of the area in which this experiment was conducted. Water is a limiting resource for plant growth in such conditions in non-irrigated agriculture [45] ; therefore, it is under these conditions that the beneficial ecosystem services, especially water infiltration into the soil [46] , would be expected to result in an increase in crop yield. This phenomenon might explain why no-tillage fields have been reported to produce higher yields than conventional tillage fields in lower rainfall years in Mediterranean environments [47] . It may be that this phenomenon is less important in wetter habitats, because water is not as limiting to plant growth and therefore to crop yield. Is it possible to capture the ecosystem service benefits created by ants and termites in agriculture in dry and hot climates, as has occurred for earthworms in wet and cool ones? There is evidence that traditional agriculture in tropical West Africa does already, as people place plant mulch and wood onto degraded soil to increase termite activity, and thereby improve the soil for cultivation [48] , [49] . Traditional agricultural knowledge is not well known outside their traditional cultures [50] , and scaling from 1-ha traditional farms to thousands of hectares in intensive agriculture may prove difficult. Lessons may be learnt from managing earthworms in agriculture; these mostly follow 'conservation agriculture' management for reducing erosion, such as reduced tillage, controlled traffic and reduced use of pesticides. The farm on which the experiment was run uses some conservation agriculture management methods and has a diverse ant and termite community; therefore, it seems likely that these methods will prove beneficial to the soil macrofauna communities in other dry and hot climates as well. The shallow tillage used as mechanical weed control did not appear to affect the soil insects or their effect on crop yield, indicating that shallow tillage may be used without damaging soil fauna. This will increase environmental sustainability while increasing economic sustainability by reducing inputs and increasing yields [2] , [7] , [8] , [9] , [10] , [11] , [12] . Clearly, these low-impact management methods will benefit soil macrofauna already found on the farm. There remains the issue of how farms without ants and termites, due to decades of intensive tillage and pesticide application, can acquire them. This is a non-trivial issue, given the size of intensively managed farms, the sometimes very low portion of land with native vegetation communities and fragmentation of such habitat [4] , [11] , [51] , which even then can have degraded ant and termite communities [52] . The results may become relevant in the future to areas predicted to become hotter and drier under climate change. Annual rainfall is predicted to decrease between 30 and 180 mm in subtropical and warm temperate latitudes, resulting in a decrease of up to 20% soil moisture [53] , especially with Mediterranean and savanna climates, and including areas used to grow cereal crops such as wheat [31] . Regions most likely to experience these changes include Northern Africa (Morocco to Egypt), Southern Africa (South Africa to Botswana), Southwest Asia (Turkey to Azerbaijan), Southern Australia, Southern Europe (Spain to Greece), Southwest North America (Panama to California) and southern South America (Chile) [53] , [54] . Future cereal production has many pressing issues, including erosion and nitrogen availability [2] , [3] , [4] , [5] , [6] , [55] , [56] , in addition to climate change; perhaps, capturing the ecosystem services provided by ants and termites will help reduce future unpredictability of food supply [1] , [2] , [7] , [8] , [12] , [55] , [56] . Questions about specific details remain to be investigated. These include whether some species or functional groups were more important than others. Earthworms are grouped according to their foraging and ecology, which affects tunnel structure and thus water infiltration in soil. The highest water infiltration is in soil with endogeic (soil foraging and soil dwelling) species and anecic (surface foraging and soil dwelling) species; the lowest is with epigeic (surface foraging and surface dwelling) species [13] , [14] , [57] . Our exclusion results may suggest that insects with differing foraging patterns affect water infiltration differentially. The higher water infiltration in control plots may have been due to surface foraging ants (such as Melophorus , Meranoplus , Monomorium and Pheidole ) and grass-harvesting termites ( Amitermes and Drepanotermes ) that live in the soil, creating an opening to the soil surface similar to anecic earthworms. In comparison, exclusion plots had some wood-feeding termites that were feeding in deeper soil on the roots of the felled trees and shrubs of the original native vegetation, as they were not affected by the insecticide. As these termites were foraging and dwelling deeper in the soil, their tunnels did not open to the soil surface, and hence correspond to the lower water infiltration. The nitrogen cycle remains to be investigated in detail, including the mechanisms of fixation, mineralization, immobilization and denitrification in the microbe community and in the micro-, meso- and macrofauna communities [36] . Such information is likely to lead to improved management for ecosystem services in dryland cropping. Field site The experiment was located in a field (27.921°S, 115.028°E) 5 km from the northeastern limits of wheat production in the west of Australia. Average annual temperatures are 13.4 °C (min) and 27.3 °C (max) and average annual rainfall is 284 mm (predominantly in winter)—close to the hottest and driest for wheat in Australia [31] . The nutrient-poor, deep sandy soil is classified (USDA Soil Taxonomy) as a Dystric Xerosamment. The natural vegetation community includes Eucalyptus , Acacia and Banksia species. The area was cleared for farming in 1980 and was managed conventionally until 2000. Concern about erosion and soil heath prompted adoption of no/low tillage, defined vehicle routes across fields (commonly known as 'controlled traffic') and stubble retention (that is, left in the field). These management methods promote the presence of ants and termites, as soil disturbance by tillage is minimized, soil is not compressed and stubble remains as a food resource. The rotation is wheat/fallow/wheat; fallow years are used, in part, to accumulate water. The farmed land supported ant species of the genera Cardiocondyla , Iridomyrmex , Melophorus , Meranoplus , Monomorium , Pheidole , Rhytidoponera , and Tetramorium and termite species of the genera Amitermes , Drepanotermes , Macrognathotermes , Microcerotermes and Nasutitermes . These species were probably absent from the field during the 20 years of conventional farm management, as they are absent from nearby fields that are still under conventional farm management. Experiment installation The experiment was a two-way factorial design, with insect exclusion and tillage as treatments. There were five replicate plots (27 m×27 m, size determined by the defined vehicle routes and ant and termite foraging behaviour) of each treatment combination. We excluded insects with a synthetic pyrethroid insecticide (FMC Biflex Ultra Emulsion, FMC; active ingredient bifenthrin, applied as per label instructions for termite barrier pre-construction treatments—3.75 g per 5 l water per m 2 ). Synthetic pyrethroids have slight and short-term effects ( ∼ 4 weeks) on soil microflora [58] . Each plot received 3,645 l of prepared insecticidal solution. This volume of water is required for the insecticide to penetrate to at least 50 mm depth, as per Australian Standard for pest subterranean termite management AS3660.1 (but likely to have infiltrated 100 mm depth based on penetration of equivalent volume rainfall events of 5 mm). We controlled for the application of the insecticide by applying 3,645 l of water to the control plots. We applied the insecticide solution and water using a truck with water tank and polyvinyl chloride pipe rigging adapted to spray water to mimic rain. Tillage was added as a second treatment because the farmer used shallow weed tillage to control summer weeds [22] , but did not know the effect of this on soil insects. The tillage was shallow, ∼ 15 cm deep, using a Grizzly 92, Sandgroper two-way tandem disc plough. For no-tillage, the plough was lifted above the soil when the tractor crossed the plot. There was only a minimal presence of weeds when the experiment was started, and there were no outbreaks of either weeds or insect herbivorous pests during the experiment. Crop management Crops were sown on 29 May 2006 and on 30 May 2008, and harvest occurred on 1 November 2006 and on 11 November 2008. The same wheat variety was used in both years. Fertilizer (di-ammonium phosphate compound) was applied uniformly at sowing across the entire field, and was not applied during the experiment. Neither insecticide nor herbicide was applied to the field during the cropping years of 2006 and 2008. Effect of exclusion We measured the effect of the exclusion by monitoring ant nests and termite foraging activity. Four people counted active ant nests by careful searching pre-treatment in May 2006 (before sowing) and post-treatment in November 2006 (immediately before harvest). We assessed termite survival by baiting. We placed six baits (one 15×20×1 cm 3 piece of Eucalyptus regnans wood, one unbleached toilet paper roll and a string bag of 20×30 cm 2 filled with stubble cut from the surrounding paddock) under a 50×50 cm 2 piece of moisture membrane) in each plot from January to June in 2008. Crop yield We measured wheat yield by collecting the grain heads from all plants encountered along replicate 1-m-long rods placed haphazardly in each plot from the two harvests (November 2006 and 2008). We collected six and ten replicate samples per plot in 2006 and 2008, respectively. We threshed the heads, dry weighed the grain and then screened the grain for small (pinched) kernels, which form due to a lack of water [59] . We converted the raw data (grain weight, g m −1 ) to variation from annual average yield (grain weight, t ha −1 ). We analysed yield in a repeated measures two-way analysis of variance (ANOVA) with log-transformed data (to improve homogeneity of variances). Because the time and exclusion interaction was significant in a repeated measures two-way ANOVA, we analysed the years separately. Insect tunnels We measured insect tunnel density after harvesting in both years by counting insect tunnels in pits (2 m long×1 m wide×2 m deep). We excavated one hole in a single plot from each treatment combination in November 2006 (to avoid the disturbance to all plots) and excavated one hole in each plot in November 2008 ( Supplementary Fig. S4a ). We recorded data from 15 to 30 quadrats (10 cm×10 cm) placed on the vertical side walls of each hole, between 10 and 50 cm deep (we could not count tunnels in the dry and crumbling soil 0–10 cm deep) ( Supplementary Fig. S4b ), depending on the condition of the soil. We analysed data using a one-way ANOVA on log-transformed data (to improve homogeneity of variance). Water infiltration We continuously monitored the rainfall and soil moisture in real time from the installation of the experiment (May 2006) until the second harvest (November 2008). We used an electronic rain gauge to measure rain every minute during rainfall and capacitance probes (Easy Ag series 2, Sentek) with sensors at 0.1, 0.2, 0.3 and 0.5 m below the soil surface to measure soil water content. There was one probe per plot in four of the replicate plots for each treatment combination. Probes were linked to data loggers, which recorded soil moisture automatically each day at 00.00 hours on days when no rain fell, and at every 15 min when rain was recorded in the rain gauge. We chose two nearly identical rain events on 8 September 2006 and 9 June 2008 to analyse increases in soil moisture. Both these specific events occurred within the cropping phase of the project and were nearly identical in rainfall volume and duration, and were preceded and followed by at least 3 days without rain. We analysed soil moisture at the maximum depth of 0.5 m deep using two-way ANOVA, years analysed separately. Soil nitrogen We sampled soil with augers (diameter 5 cm) to 0.5 m depth immediately after harvest in 2006 and 2008. Soil from 0 to 10 cm depth was analysed for mineral nitrogen content in a commercial laboratory (CSBP Soil and Plant Analysis Laboratory, Bibra Lake Western Australia). The soil nitrate nitrogen and ammonium nitrogen were extracted with a 1 M KCl solution for 1 h at 25 °C. The resulting soil solution was diluted and measured on a Lachat Flow Injection Analyzer. The concentration of ammonium nitrogen was measured colorimetrically at 420 nm using the indo-phenol blue reaction. Nitrate was reduced to nitrite through a copperized cadmium column, and the nitrite was also measured colorimetrically at 520 nm. Ammonium and nitrate behaved similarly during both times of measurement; hence, we calculated total soil mineral nitrogen as ammonium plus nitrate, and analysed total mineral nitrogen in a repeated measures two-way ANOVA with log-transformed data (to improve homogeneity of variance). The repeated measures two-way ANOVA showed that the year × exclusion interaction was significant; hence, we analysed the data from each year separately using two-way ANOVAs. Nitrogen fixation genes in termite gut flora We collected termites haphazardly from the plots during the experimental installation in May 2006, and stored them in 100% ethanol. We chose Coptotermes sp. and Drepanotermes sp., as they were the most phylogenetically distant genera sampled and they eat different foods (sound wood and dead grass, respectively). We used worker termites for each species, washed them in distilled water, removed their guts and separated the gut contents by gentle squeezing. The DNA in the gut contents was then purified with an Accuprep DNA extraction kit (Bioneer). We followed published methods for detection of 406 bp of the nifH gene [34] . We amplified nifH genes using PCR, then cloned the PCR products and sequenced two clones from the Coptotermes sample and four clones from the Drepanotermes sample using a commercial sequencing service (Macrogen, South Korea). We then performed Blast on the six clones; the top ten hits retrieved for each clone were nifH genes from uncultured termite gut bacteria (nucleotide identity levels of 82–88%). How to cite this article: Evans, T.A. et al . Ants and termites increase crop yield in a dry climate. Nat. Commun. 2:262 doi: 10.1038/ncomms1257 (2011).